Absence of surrogate light chain results in spontaneous autoreactive germinal centres expandingVH81X-expressing B cells Random recombination of antibody heavy- and light-chain genes results in a diverse B-cell receptor (BCR) repertoire including self-reactive BCRs. However, tolerance mechanisms that prevent the development of self-reactive B cells remain incompletely understood. The absence of the surrogate light chain, which assembles with antibody heavy chain forming a pre-BCR, leads to production of antinuclear antibodies (ANAs). Here we show that the naive follicular B-cell pool is enriched for cells expressing prototypic ANA heavy chains in these mice in a non-autoimmune background with a broad antibody repertoire. This results in the spontaneous formation of T-cell-dependent germinal centres that are enriched with B cells expressing prototypic ANA heavy chains. However, peripheral tolerance appears maintained by selection thresholds on cells entering the memory B-cell and plasma cell pools, as exemplified by the exclusion of cells expressing the intrinsically self-reactive V H 81X from both pools. Autoimmune diseases, for example, systemic lupus erythematosus (SLE) and rheumatoid arthritis (RA), have been associated with defective B-cell tolerance, mechanisms that in healthy individuals prevent the development of self-reactive naive peripheral B cells [1] , [2] , [3] . A hallmark of these diseases is the production of autoantibodies [4] , [5] , for instance, anti-DNA and antinuclear antibodies (ANAs) in SLE, which can be detected long before disease onset [6] , [7] . Autoantibodies are produced under both T-cell-independent and -dependent (Td) conditions. The latter are of particular concern as they involve germinal centre (GC) formation, secondary structures that support B-cell clonal expansion, alter antibody effector function and antigen affinity, and result in immunological memory that can last for a lifetime [8] , [9] , [10] , [11] , [12] . In autoimmune diseases, and mouse models thereof, GCs develop spontaneously [13] , [14] , suggesting additional levels of self-tolerance acting at GCs that are defective in these diseases [15] . Random recombination of V(D)J gene segments, encoding antibody heavy and light chain variable regions, results in a highly diverse primary repertoire of B-cell receptors (BCRs), that is, membrane-bound antibodies. As the recombination also results in those that are self-reactive, several mechanisms are in place to eliminate self-reactivity from the naive B-cell pool. At the pro-B-cell stage early in B-cell development VDJ H recombination leads to expression of an antibody μ-heavy (μH) chain. This assembles with the invariant surrogate light (SL) chain, encoded by VpreB and λ5 , and the signalling molecules Igα/β forming a pre-BCR [16] , [17] , where association with the SL chain serves as a quality control of μH chains. A dysfunctional μH chain results in a block in B-cell development at the pro-B-cell stage, whereas a dysfunctional SL chain allows these cells to transit to the pre-B-cell stage, although pre-B-cell numbers are greatly reduced [16] . The H chain complementarity determining region 3 (H-CDR3), encoded by the V H DJ H junction, is the most variable of the three CDRs, and plays a central role in recognition of both antigen and autoantigen [18] , [19] , [20] , [21] , [22] , [23] . A characteristic of a majority of anti-DNA and ANAs is a H-CDR3 with one, or more, basic amino acid (aa) residues (ANA H-CDR3) that is critical to antigen binding [15] , [21] . Also the non-Ig portion of λ5 (λ5-tail) contains basic amino acid residues that are critical to pre-BCR signalling [24] , [25] , [26] , [27] . Moreover, some of the pre-B cells that develop in both mice and humans with a dysfunctional SL chain [28] , [29] express μH chains characterized by a prototypic ANA H-CDR3 (refs 24 , 25 ). Nevertheless, as the pre-B cells in mice lacking SL chain ( SLC −/− ) proceed in development, they encounter strong selection pressure as both immature and transitional B cells [30] . Despite this B-cell tolerance is seemingly defective, as serum levels of, for example, anti-double-stranded DNA and ANAs are elevated in these mice [28] . SL chain is only expressed in early B-cell lineage cells, and hence its absence represents a monogenic and B-cell intrinsic defect. The SLC −/− mouse is thus a unique model in which to investigate B-cell tolerance mechanisms without the complexity of multiple genetic loci being involved, as in multigenic autoimmune diseases. Moreover, as they express a diverse antibody repertoire and on a lupus-resistant background, this model allows the changes in the BCR repertoire imposed by tolerance mechanisms to be uncovered not possible with monoclonal Ig transgenic mice. Using the SLC −/− mouse model, we have investigated whether self-reactive naive peripheral B cells develop and the consequences of this. We show that the pool of naive B cells in SLC −/− mice is indeed enriched for autoreactivity, and that this in itself is sufficient to initiate spontaneous formation of persistent Td GCs. However, peripheral tolerance appears maintained by selection thresholds on GC B cells entering the memory B-cell and plasma cell pools. B cells with prototypic ANA H-CDR3 enriched in SLC −/− mice To investigate whether self-reactive naive follicular (FO) B cells develop in SLC −/− mice, we used a prototypic ANA H-CDR3 (1 or ≥2 arginine and/or lysine) as a marker. Assessing μH chains expressed during B-cell development, we observed a decrease in proportions of cells with a prototypic ANA H-CDR3 comparing pro-B with FO B cells from control mice ( P <0.0001; χ 2 -test; Fig. 1a ). By contrast, in SLC −/− mice, an enrichment was evident in the pre-B compared with the pro-B cells ( P <0.0001; χ 2 -test), and in the immature B cells the proportions were even higher ( P <0.0001; χ 2 -test), where a majority of H-CDR3 contained one arginine/lysine. In the FO B cells, a reduction was observed compared with the immature B (and pre-B) cells ( P <0.0001; χ 2 -test), however, the proportions of both those with 1 and ≥2 arginine and/or lysine were still higher in the FO B cells from SLC −/− mice than in controls ( P <0.0001; χ 2 -test). Thus, cells that express μH chains with a prototypic ANA H-CDR3 are enriched in SLC −/− mice among pre-B cells, as well as at later developmental stages, consistent with the notion that the pool of naive FO B cells in SLC −/− mice is enriched for autoreactivity. 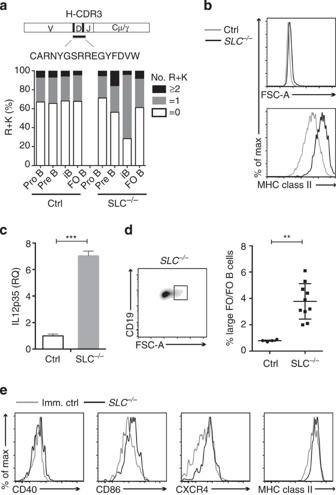Figure 1: FO B cells with prototypic ANA H-CDR3 are enriched inSLC−/−mice, and includes a subset of large, activated cells. (a) Sequence analysis of Ig μH chains expressed in pro-B (14610; 12906), pre-B (12870; 1950), immature B (35516; 9152) and FO B (29554; 564) cells in control (Ctrl) andSLC−/−mice, showing proportions of H-CDR3 sequences with 0, 1 or ≥2 arginine (R) and/or lysine (K) residues. (b,d,e) Flow cytometry analysis of spleen cells. (b) Expression of indicated parameters on FO B cells from Ctrl andSLC−/−mice. (c) QPCR analysis ofIL12p35in FO B cells from indicated mice. The mRNA levels were normalized to β-actin. Levels in FO B cells from Ctrl mice were set to 1. (d) Gating on FO B cells fromSLC−/−mice plot shows forward scatter (FSC) versus CD19, indicating a subset of cells that is larger in cellular size. Graph shows % large cells of total FO B cells in Ctrl andSLC−/−mice. (e) Histograms show expression of indicated markers on the subset of larger FO B cells inSLC−/−and SRBC-immunized (Imm.) ctrl mice. Data inaare from a pool of six mice. Numbers in parenthesis indicate unique sequences from ctrl andSLC−/−mice, respectively. Data (b–e) are representative or pooled (c) from at least two independent experiments. Each symbol represents one mouse. Error bars represent s.e.m.Pvalues were determined using a two-tailedt-test. **P<0.01, ***P<0.001. Figure 1: FO B cells with prototypic ANA H-CDR3 are enriched in SLC −/− mice, and includes a subset of large, activated cells. ( a ) Sequence analysis of Ig μH chains expressed in pro-B (14610; 12906), pre-B (12870; 1950), immature B (35516; 9152) and FO B (29554; 564) cells in control (Ctrl) and SLC −/− mice, showing proportions of H-CDR3 sequences with 0, 1 or ≥2 arginine (R) and/or lysine (K) residues. ( b , d , e ) Flow cytometry analysis of spleen cells. ( b ) Expression of indicated parameters on FO B cells from Ctrl and SLC −/− mice. ( c ) QPCR analysis of IL12p35 in FO B cells from indicated mice. The mRNA levels were normalized to β-actin. Levels in FO B cells from Ctrl mice were set to 1. ( d ) Gating on FO B cells from SLC −/− mice plot shows forward scatter (FSC) versus CD19, indicating a subset of cells that is larger in cellular size. Graph shows % large cells of total FO B cells in Ctrl and SLC −/− mice. ( e ) Histograms show expression of indicated markers on the subset of larger FO B cells in SLC −/− and SRBC-immunized (Imm.) ctrl mice. Data in a are from a pool of six mice. Numbers in parenthesis indicate unique sequences from ctrl and SLC −/− mice, respectively. Data ( b – e ) are representative or pooled ( c ) from at least two independent experiments. Each symbol represents one mouse. Error bars represent s.e.m. P values were determined using a two-tailed t -test. ** P <0.01, *** P <0.001. Full size image A subset of pre-GC B cells among the naive FO B-cell pool Next we investigated whether the apparent lack of tolerance among FO B cells in SLC −/− mice was accompanied by a change in phenotype. The FO B cells from these mice were larger in size and the levels of major histocompatibility complex (MHC) class II were higher ( Fig. 1b ), whereas those of IgM, IgD, CD19, CD40, CD69 and CD23 were not changed to the same extent or not at all ( Supplementary Fig. 1a ). Although this could indicate a state of activation, the levels of p-Erk or p-Blnk were not elevated ( Supplementary Fig. 1b ). Microarray analysis of RNA from FO B cells showed that the levels of Fas and Cd40 , and those of Ccl3 and Ccl5 (encoding chemokines) were higher in the FO B cells from SLC −/− mice than controls ( Supplementary Table 1 ). Most noticeable were the elevated levels of IL-12a , a cytokine that supports differentiation into T follicular helper (T FH ) cells [31] , which was confirmed by quantitative PCR (qPCR) of IL12p35 ( Fig. 1c ). We also noticed that the FO B cells from SLC −/− mice could be divided into two subsets based on cellular size ( Fig. 1d ). The proportion of large cells was increased compared with controls already at an age of 4–5 weeks, and also at this age the larger cells expressed higher levels of CD86 and MHC class II ( Supplementary Fig. 2a–c ). Together, these data suggest that a subset of the FO B cells in SLC −/− mice is activated, and that this involves signalling through the BCR and toll like receptor (TLR) ( Ccl3 and Ccl5 ) pathways [32] , [33] , as well as interactions with T cells. Because of the apparent involvement of T cells in activating the FO B cells, to generate B cells typical of Td immune responses for comparison, we immunized control mice with sheep red blood cells (SRBCs). One and two weeks post immunization, a subset of larger cells was detected among the splenic FO B cells with higher levels of CD40, CD86, CXCR4 and MHC class II than on the small cells ( Supplementary Fig. 3 ). The size of these large cells in the immunized control mice was similar to that of the larger FO B cells in (unimmunized) SLC −/− mice, as were the levels of CD40, CD86, CXCR4 and MHC class II ( Fig. 1e ). Over the last years, precursors of GC (pre-GC) B cells have been described [34] , which opened the possibility that the large FO B cells in SLC −/− mice represented pre-GC B cells. Spontaneous formation of GCs The uncovering of potential pre-GC B cells in SLC −/− mice prompted us to investigate whether we could also detect GCs. Analysing splenic cryosections identified B220 + GL7 + cells located in B-cell follicles close to the T:B-cell border in SLC −/− mice but not in control mice ( Fig. 2a ), and flow cytometry analysis confirmed the presence of a CD19 + CD95 + GL7 + B-cell population in SLC −/− mice ( Fig. 2b,c ). Thus, GCs develop spontaneously in SLC −/− mice, an unexpected observation, considering that the mice had not been actively immunized. Investigating the kinetics showed that in 4-week-old SLC −/− mice, few, if any, GCs were detected by contrast to 7–8-week-old mice when GCs were found in ∼ 70% of the animals, and by 10–14 weeks nearly all mice presented with GCs ( Fig. 2d,e ). Their presence also at an age of 30–35 weeks suggested that in SLC −/− mice, the GCs persist over long periods of time. 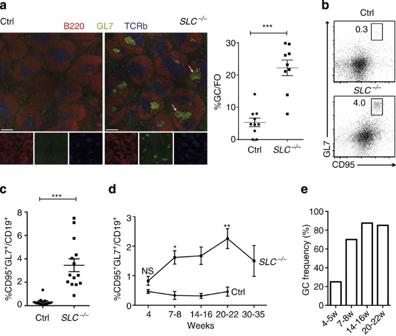Figure 2: Spontaneous formation of splenic GCs. (a) Immunofluorescence staining of spleen cryosections from control (Ctrl) andSLC−/−mice. GL7 (green), B220 (red) and TCRβ (blue). Arrows indicate GC structures, × 10 objective; scale bars, 200 μm. Graph shows % GCs per follicles (FO, two independent observers). (b–e) Flow cytometry analysis of spleen cells. (b) Dot plots show CD95+GL7+GC B cells among CD19+B cells. (c) Graph shows % CD95+GL7+GC B cells among CD19+B cells in Ctrl andSLC−/−mice. (d) Graph shows % CD95+GL7+cells in CD19+B cells at indicated ages in Ctrl andSLC−/−mice. (e) Graph shows frequency of mice with ≥1.0% CD95+GL7+cells in CD19+B cells at indicated ages inSLC−/−mice. Data inaandbare representative, and inaandc–eare pooled from at least two independent experiments. Each symbol represents one mouse. Error bars represent s.e.m.Pvalues were determined using a two-tailedt-test. *P<0.05; **P<0.01; ***P<0.001; NS, not significant; w, weeks. Figure 2: Spontaneous formation of splenic GCs. ( a ) Immunofluorescence staining of spleen cryosections from control (Ctrl) and SLC −/− mice. GL7 (green), B220 (red) and TCRβ (blue). Arrows indicate GC structures, × 10 objective; scale bars, 200 μm. Graph shows % GCs per follicles (FO, two independent observers). ( b – e ) Flow cytometry analysis of spleen cells. ( b ) Dot plots show CD95 + GL7 + GC B cells among CD19 + B cells. ( c ) Graph shows % CD95 + GL7 + GC B cells among CD19 + B cells in Ctrl and SLC −/− mice. ( d ) Graph shows % CD95 + GL7 + cells in CD19 + B cells at indicated ages in Ctrl and SLC −/− mice. ( e ) Graph shows frequency of mice with ≥1.0% CD95 + GL7 + cells in CD19 + B cells at indicated ages in SLC −/− mice. Data in a and b are representative, and in a and c – e are pooled from at least two independent experiments. Each symbol represents one mouse. Error bars represent s.e.m. P values were determined using a two-tailed t -test. * P <0.05; ** P <0.01; *** P <0.001; NS, not significant; w, weeks. Full size image Splenic GCs are present after antibiotics treatment The spontaneous formation of GCs in SLC −/− mice was unexpected, as they had not been actively immunized and the defect is B-cell intrinsic. However, as the FO B cells in these mice were enriched for cells expressing a BCR with a prototypic ANA H-CDR3, we reasoned that a possible trigger for GC formation could have been the gut microbiota, as a germ-free environment has been shown to lead to milder disease in some autoimmune models [35] . To investigate the influence of intestinal microbes, SLC −/− mice were placed on broad-spectrum antibiotics from the time of weaning, when GCs had not yet been established ( Fig. 2d ), in order to deplete of the normal gut microbiota ( Fig. 3a ). As expected from this treatment [36] , the proportion of GC B cells in Peyer’s patches were reduced in SLC −/− mice treated with antibiotics ( Fig. 3b,c ), which was corroborated by a reduction in IgA plasma cells in the intestine and faecal bacterial load ( Fig. 3d,e ). In the antibiotic, but not untreated, group, the spleen size was much smaller as shown by the reduction in B-cell numbers ( Fig. 3f ). However, the proportion of splenic GC B cells was not changed ( Fig. 3g ), which was corroborated by the presence of GC structures and serum IgG ANAs in both groups ( Supplementary Tables 2 and 3 ). It would thus appear that the gut microbiota is not the main trigger of GC formation in SLC −/− mice. 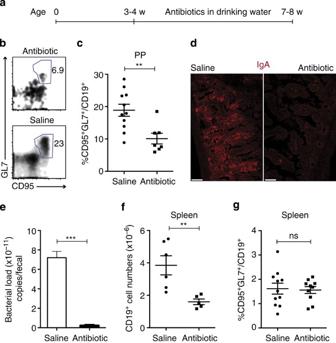Figure 3: Gut microbiota is not a main trigger of spontaneous GC formation. (a–g)SLC−/−mice were treated with broad-spectrum antibiotics or saline water. (a) Experimental design: antibiotic treatment ofSLC−/−mice was started at an age of 3–4 weeks (w) and completed 4 weeks later. (b) Dot plots show CD95+GL7+cells in CD19+cells from Peyer’s patches (PP). (c) Graph shows % of CD95+GL7+cells in CD19+cells from PP. (d) Immunofluorescence staining of intestine cryosections with antibodies detecting IgA, × 10 objective; scale bars, 50 μm. (e) qPCR analysis of total bacterial DNA copy numbers in faeces. (f) Graph shows total splenic CD19+cell numbers. (g) Graph shows % splenic CD95+GL7+cells among CD19+cells. Data are representative from two independent experiments. Each symbol represents one mouse. Error bars represent s.e.m.Pvalues were determined using a two-tailedt-test. **P<0.01, ***P<0.001; NS, not significant. Figure 3: Gut microbiota is not a main trigger of spontaneous GC formation. ( a – g ) SLC −/− mice were treated with broad-spectrum antibiotics or saline water. ( a ) Experimental design: antibiotic treatment of SLC −/− mice was started at an age of 3–4 weeks (w) and completed 4 weeks later. ( b ) Dot plots show CD95 + GL7 + cells in CD19 + cells from Peyer’s patches (PP). ( c ) Graph shows % of CD95 + GL7 + cells in CD19 + cells from PP. ( d ) Immunofluorescence staining of intestine cryosections with antibodies detecting IgA, × 10 objective; scale bars, 50 μm. ( e ) qPCR analysis of total bacterial DNA copy numbers in faeces. ( f ) Graph shows total splenic CD19 + cell numbers. ( g ) Graph shows % splenic CD95 + GL7 + cells among CD19 + cells. Data are representative from two independent experiments. Each symbol represents one mouse. Error bars represent s.e.m. P values were determined using a two-tailed t -test. ** P <0.01, *** P <0.001; NS, not significant. Full size image Skewed ratio of T FH to GC B cells GC formation and maintenance is controlled by the interplay between different cell types, including follicular dendritic cells (FDCs), T FH cells and B cells [37] , [38] , [39] , [40] , [41] , [42] . In SLC −/− mice, networks of CD35 + FDCs were detected in the GC zone proximal to the B-cell follicle ( Fig. 4a ); most likely in the light zone (LZ) where B cells would normally encounter FDC-trapped antigens. Assessing the presence of T cells demonstrated that TCRβ + cells were located in the GCs ( Fig. 2a ), as well as CD4 + cells of which some were Bcl-6 + ( Fig. 4b ), the pivotal transcription factor expressed by T FH cells. The presence of T FH cells in SLC −/− mice was confirmed by the enrichment of CD4 + cells expressing high levels of PD-1 ( Fig. 4c,d ), whereas number of CD4 + T cells as well as percentage of regulatory T cells within this pool were similar in SLC −/− and control mice ( Supplementary Fig. 4a,b ). Moreover, CD62L, a cell adhesion molecule that is downregulated upon activation of naive CD4 + T cells, was absent on the vast majority of CD4 + PD-1 hi cells by contrast to most CD4 + cells ( Fig. 4e ). Analyses by qPCR confirmed the expression of Bcl6 , and demonstrated high levels of Cxcr5 in CD4 + PD-1 hi compared with CD4 + PD-1 − cells ( Fig. 4f ). This assay also showed higher levels of Il4 , Ifng and Tbx21 (T-bet), as well as a 1,000-fold increase in Il21 mRNA levels in the CD4 + PD-1 hi population but unchanged levels of Tgfb1 . 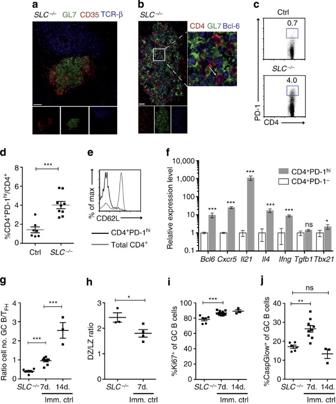Figure 4: Skewed ratio of TFH:GC B cells. (a,b) Immunofluorescence staining of spleen cryosections fromSLC−/−mice. GL7 (green). (a) Detection of CD35+FDC networks. CD35 (red), TCRβ (blue), × 25 objective; scale bar, 50 μm. (b) Detection of CD4+TFHcells, and those expressing Bcl-6 (arrow). CD4 (red), Bcl-6 (blue), × 40 objective; scale bar, 20 μm. (c–e,g–j) Flow cytometry analysis of spleen cells. (c) CD4+PD-1hiTFHcells gated on CD4+cells in Ctrl andSLC−/−mice. (d) Graph shows percentages CD4+PD-1hiTFHcells gated on CD4+cells. (e) Expression of CD62L on CD4+and CD4+PD-1hiT cells fromSLC−/−mice. (f) QPCR analysis ofBcl6,Cxcr5,Il21,Il4,Ifng,Tgfb1andTbx21(T-bet) mRNA levels in naive CD4+PD-1−and CD4+PD-1hiT cells fromSLC−/−mice, with β-actin as internal ctrl. (g) Graph shows ratio of GC B/TFHcell numbers inSLC−/−and SRBC-immunized control (Imm. ctrl) mice. (h) Graph shows DZ/LZ ratio in indicated genotypes. (i) Graph shows % Ki-67+cells in the CD19+CD95+GL7+gate. (j) Graph shows % CaspGlow+(activated caspases) in the CD19+CD95+GL7+gate. Data are representative from at least two independent experiments except for (g,i,j) day (d) 14 post immunization, which was only performed once. Data indare pooled from three independent experiments. Each symbol represents one mouse. Data infare from two independent experiments with at least four mice in each. Error bars represent s.e.m.Pvalues were determined using a two-tailedt-test. *P<0.05, **P<0.01, ***P<0.001; NS, not significant. Figure 4: Skewed ratio of T FH :GC B cells. ( a , b ) Immunofluorescence staining of spleen cryosections from SLC −/− mice. GL7 (green). ( a ) Detection of CD35 + FDC networks. CD35 (red), TCRβ (blue), × 25 objective; scale bar, 50 μm. ( b ) Detection of CD4 + T FH cells, and those expressing Bcl-6 (arrow). CD4 (red), Bcl-6 (blue), × 40 objective; scale bar, 20 μm. ( c–e , g – j ) Flow cytometry analysis of spleen cells. ( c ) CD4 + PD-1 hi T FH cells gated on CD4 + cells in Ctrl and SLC −/− mice. ( d ) Graph shows percentages CD4 + PD-1 hi T FH cells gated on CD4 + cells. ( e ) Expression of CD62L on CD4 + and CD4 + PD-1 hi T cells from SLC −/− mice. ( f ) QPCR analysis of Bcl6 , Cxcr5 , Il21 , Il4 , Ifng , Tgfb1 and Tbx21 (T-bet) mRNA levels in naive CD4 + PD-1 − and CD4 + PD-1 hi T cells from SLC −/− mice, with β-actin as internal ctrl. ( g ) Graph shows ratio of GC B/T FH cell numbers in SLC −/− and SRBC-immunized control (Imm. ctrl) mice. ( h ) Graph shows DZ/LZ ratio in indicated genotypes. ( i ) Graph shows % Ki-67 + cells in the CD19 + CD95 + GL7 + gate. ( j ) Graph shows % CaspGlow + (activated caspases) in the CD19 + CD95 + GL7 + gate. Data are representative from at least two independent experiments except for ( g , i , j ) day (d) 14 post immunization, which was only performed once. Data in d are pooled from three independent experiments. Each symbol represents one mouse. Data in f are from two independent experiments with at least four mice in each. Error bars represent s.e.m. P values were determined using a two-tailed t -test. * P <0.05, ** P <0.01, *** P <0.001; NS, not significant. Full size image As expected, T FH cells were also detected in the SRBC-immunized control mice ( Fig. 4g ). However, as the number of T FH but not GC B cells was similar in SLC −/− and immunized control mice, the ratio of T FH to GC B cells differed ( Fig. 4g ). In the immunized control mice, the ratio changed such that at 1 week into the response it was 1:1, whereas at 2 weeks there were less T FH cells per GC B cells (1:2.5). By contrast, in SLC −/− mice, the ratio was reversed with more T FH cells per GC B cells (2:1), hence fivefold more compared with the SRBC response at 2 weeks. Thus, the cellular composition in the spontaneously developing GCs in SLC −/− mice is altered. Reduced expansion and apoptosis of GC B cells T FH cells are pivotal to GC B-cell dynamics providing signals affecting their expansion, survival and fate [37] , [38] , [39] , [42] , [43] , [44] . GCs can be divided into dark zone (DZ) and LZ, with B-cell proliferation taking place in the former and selection in the latter, where T cells and FDCs are mainly located. Determining the ratio of DZ:LZ, based on surface expression of CXCR4 and CD86, showed that this was 2.3:1 in SLC −/− mice and 1.8:1 in SRBC-immunized control mice ( Fig. 4h ). The proportion of GC B cells that expressed the proliferation marker Ki-67 was lower in SLC −/− mice than in immunized controls, 80% and 90%, respectively ( Fig. 4i ). The expression of Ki-67 in SLC −/− GCs was confirmed on cryosections ( Supplementary Fig. 5a ). Staining for active caspases, a marker of cells prone to undergoing apoptosis showed that the proportions in SLC −/− mice were about the same as those in immunized control mice at 2 weeks but not at 1 week ( Fig. 4j ). Moreover, splenic GC B cells in SLC −/− mice expressed Bcl-6 ( Fig. 4b and Supplementary Fig. 5b ), a transcription factor critical also for GC B cells. Thus, the cellular dynamics in the spontaneously developing GCs in SLC −/− mice are altered, resulting in reduced expansion and apoptosis of the GC B cells. B:T-cell interactions are required for maintenance of pre-GC B cells and GCs To address whether T cells were required for GC maintenance in SLC −/− mice, the CD40:CD40L co-stimulation, necessary for cognate B:T-cell interactions [37] , [38] , [39] , [45] , was disrupted by treating the mice with anti-CD40L antibodies ( Fig. 5a ). Analyses 6 days after the first injection demonstrated that this treatment completely abolished the GC structures ( Fig. 5b and Supplementary Fig. 6a ), corroborated by the severe reduction in CD95 + GL7 + cells ( Supplementary Fig. 6b ). This effect was still evident 5 weeks after the initial injection, when GC B cells were still absent and T FH cells reduced ( Fig. 5c,d ). Moreover, the reduction in pre-GC B cells ( Fig. 5e ) also demonstrated their dependence on CD40/CD40L co-stimulation. By contrast, the proportions of FO, B1 or marginal zone B cells were not reduced 5 weeks after anti-CD40L antibody treatment ( Supplementary Fig. 6c ). Thus, the maintenance of pre-GC B cells as well as GCs in SLC −/− mice requires B:T-cell interactions. 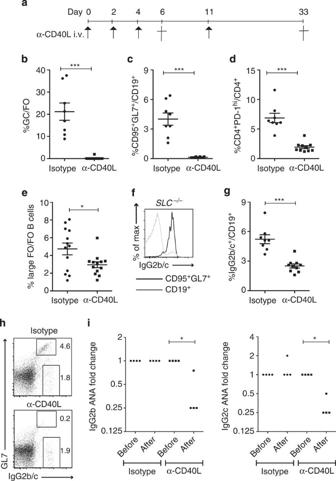Figure 5: Td maintenance of GCs and serum IgG2b/c ANAs. (a–e,g–i)SLC−/−mice were treated with anti-CD40L or isotype control antibodies, and killed after 6 days (b) or 5 weeks (c–e,g–i). (a) Experimental setup. (b) Graph shows % GCs per follicles (FO, two independent observers). (c–h) Flow cytometry analysis of spleen cells. (c) Graph shows % CD95+GL7+cells among CD19+cells. (d) Graph shows % CD4+PD-1hicells among CD4+cells. (e) Graph shows % large cells of total FO B cells. (f) Expression of cell surface IgG2b/c after gating on GL7+and CD19+cells inSLC−/−mice. Note that these are untreated. (g) % IgG2b/c+cells among CD19+cells. (h) Expression of IgG2b/c on GL7+and GL7−cell populations among CD19+cells. (i) Graphs show fold change of serum IgG2b and IgG2c ANAs before and after treatment. Data are representative and pooled (b–e,g) from at least two independent experiments. Each symbol represents one mouse. Error bars represent s.e.m.Pvalues were determined using a two-tailedt-test. *P<0.05, ***P<0.001; i.v., intravenous; NS, not significant. Figure 5: Td maintenance of GCs and serum IgG2b/c ANAs. ( a–e , g – i ) SLC −/− mice were treated with anti-CD40L or isotype control antibodies, and killed after 6 days ( b ) or 5 weeks ( c–e , g – i ). ( a ) Experimental setup. ( b ) Graph shows % GCs per follicles (FO, two independent observers). ( c – h ) Flow cytometry analysis of spleen cells. ( c ) Graph shows % CD95 + GL7 + cells among CD19 + cells. ( d ) Graph shows % CD4 + PD-1 hi cells among CD4 + cells. ( e ) Graph shows % large cells of total FO B cells. ( f ) Expression of cell surface IgG2b/c after gating on GL7 + and CD19 + cells in SLC −/− mice. Note that these are untreated. ( g ) % IgG2b/c + cells among CD19 + cells. ( h ) Expression of IgG2b/c on GL7 + and GL7 − cell populations among CD19 + cells. ( i ) Graphs show fold change of serum IgG2b and IgG2c ANAs before and after treatment. Data are representative and pooled ( b – e , g ) from at least two independent experiments. Each symbol represents one mouse. Error bars represent s.e.m. P values were determined using a two-tailed t -test. * P <0.05, *** P <0.001; i.v., intravenous; NS, not significant. Full size image Td production of serum IgG2b and IgG2c ANAs Our previous work implicated a CD21 − 23 − mature B-cell population as the origin of IgG ANA production in SLC −/− mice [28] . Here we find that the GC B cells represent a subset of this population; high levels of GL7 were expressed on 20–25% of this but not on classical B-cell populations ( Supplementary Fig. 7a,b ). Further analysis confirmed that a subset of the CD21 − 23 − population in SLC −/− mice displayed a phenotype typical of GC B cells ( Supplementary Fig. 7c ). This opened up the possibility that the GC B cells give rise to the plasma cells producing IgG ANAs in SLC −/− mice. Consistent with this, the process of class switch recombination was active in the GC B cells; the levels of Aicda , encoding the enzyme pivotal for class switch recombination, and Ig γ2b and γ2c sterile transcripts, and V J558 DJ-γ2b and - γ2c mRNA were all higher than in FO B cells from SLC −/− and control mice ( Supplementary Fig. 8a–c ). Moreover, the vast majority (90%) of GC B cells expressed IgG2b/c on their surface ( Fig. 5f ). We also detected IgG2c serum ANAs ( Supplementary Fig. 8d ) in addition to the IgG2b ANAs [28] , the former an isotype specific to Td responses, whereas the latter is produced also under T-cell-independent conditions. Investigating the effect of anti-CD40L antibody treatment showed that the absence of GC B cells 5 weeks after the initial injection correlated with a decrease in IgG2b/c-expressing GC B cells ( Fig. 5g,h ). Moreover, at this time point, serum IgG2b and IgG2c ANA levels were also reduced in SLC −/− mice treated with anti-CD40L antibodies as compared with prior treatment or isotype-treated controls ( Fig. 5i ). Thus, ANA production in SLC −/− mice is Td, and suggests that the GC B cells give rise to short-lived plasma cells producing the IgG2b and IgG2c ANAs. Development of CD80 + PD-L2 + CD73 + memory B cells Although the GC B cells gave rise to plasma cells, it was unclear whether they would give rise to memory B cells, which can be defined as CD80 + PD-L2 + CD73 + cells [46] . We could detect a CD80 + PD-L2 + subset among the splenic B cells in SLC −/− mice but not in control mice ( Fig. 6a ). These cells also expressed CD73 + , whereas the CD80 − PD-L2 − cells did not, which is consistent with memory and naive B cells, respectively. Moreover, ∼ 70% of the CD80 + PD-L2 + CD73 + cells expressed IgM ( Fig. 6b ). 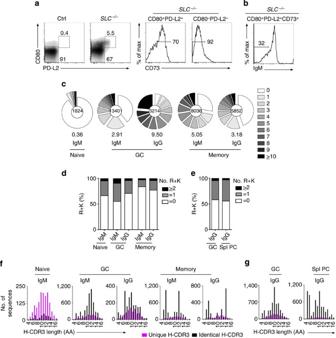Figure 6: Selection thresholds based on a prototypic ANA H-CDR3. (a,b) Flow cytometry analysis of spleen cells. (a) Plots show surface expression of CD80 and PD-L2 on B cells from control andSLC−/−mice. Plots show CD73 expression on CD80+PD-L2+and CD80−PD-L2−B cells fromSLC−/−mice. (b) Histogram shows IgM expression on CD80+PD-L2+CD73+B cells, bar indicates % IgM−cells. (c) Analysis of expressedVHDJsequences in sorted naive, GC and memory B cells. Pie charts show the proportions ofVHsequences that carry 1, 2, 3 and so on point mutations in indicated cell populations. Below is shown the average number of mutations perVH. (d,e) Proportions of H-CDR3 sequences with 0, 1 or ≥2 arginine (R) and/or lysine (K) residues in indicated cell populations. (f,g) H-CDR3 length distribution in indicated cell populations, with unique and identical sequences, pink and black bars, respectively. Data are representative from at least two independent experiments (a,b). Data are from a pool of six (c,d,f) and five (e,g)SLC−/−mice. The number of sequences analysed are at the pie chart centre. Figure 6: Selection thresholds based on a prototypic ANA H-CDR3. ( a , b ) Flow cytometry analysis of spleen cells. ( a ) Plots show surface expression of CD80 and PD-L2 on B cells from control and SLC −/− mice. Plots show CD73 expression on CD80 + PD-L2 + and CD80 − PD-L2 − B cells from SLC −/− mice. ( b ) Histogram shows IgM expression on CD80 + PD-L2 + CD73 + B cells, bar indicates % IgM − cells. ( c ) Analysis of expressed V H DJ sequences in sorted naive, GC and memory B cells. Pie charts show the proportions of V H sequences that carry 1, 2, 3 and so on point mutations in indicated cell populations. Below is shown the average number of mutations per V H . ( d , e ) Proportions of H-CDR3 sequences with 0, 1 or ≥2 arginine (R) and/or lysine (K) residues in indicated cell populations. ( f , g ) H-CDR3 length distribution in indicated cell populations, with unique and identical sequences, pink and black bars, respectively. Data are representative from at least two independent experiments ( a , b ). Data are from a pool of six ( c , d , f ) and five ( e , g ) SLC −/− mice. The number of sequences analysed are at the pie chart centre. Full size image To ensure that the CD80 + PD-L2 + CD73 + population represented memory B cells, the expressed antibody V H genes were analysed for signs of somatic hypermutation (SHM). By contrast to the naive B cells (CD80 − PDL2 − CD73 − ), where very few sequences were mutated and with <1 mutation per V H , ∼ 60% and 95% of sequences from the IgM- and IgG-expressing GC B cells were mutated with a mean of 3 and 10 mutations per V H , respectively ( Fig. 6c ). In the IgM- and IgG-expressing CD80 + PD-L2 + CD73 + population, ∼ 70% and 55% of sequences were mutated, with a mean of five and three mutations per V H , respectively. Thus, the BCRs expressed by the GC B cells and the CD80 + PD-L2 + CD73 + cells in SLC −/− mice have undergone SHM, corroborating that the latter are indeed memory B cells. A molecular basis for the spontaneous formation of GCs in SLC −/− mice By analogy to typical Td immune responses, it would appear that the GC B cells in SLC −/− mice also derived from FO B cells. However, as the GCs in SLC −/− mice developed spontaneously, the actual antigen(s) that initiated and was driving the response is unknown. Owing to the enrichment of FO B cells that expressed μH chains with a prototypic ANA H-CDR3 ( Fig. 1a ), and our observation that the GC B cells gave rise to short-lived plasma cells secreting IgG ANAs ( Fig. 5i ), this indicated ANA H-CDR3 as a potential link between the two. Investigating the H chains expressed by GC B cells, we found that those expressing IgM were indeed enriched for μH chains with prototypic ANA H-CDR3 sequences as compared with those of the naive B-cell population ( P <0.001; χ 2 -test), in fact, both those with 1 and ≥2 arginine and/or lysine ( Fig. 6d ). Thus, this provides a molecular basis for the spontaneous formation of the GCs in SLC −/− mice. Selection thresholds based on a prototypic ANA H-CDR3 Considering that a prototypic ANA H-CDR3 was an advantage among IgM-expressing GC B cells, we investigated whether we could see signs of selection in the GCs. We observed a reduction in proportions with a prototypic ANA H-CDR3 among GC B cells expressing IgG ( P <0.001; χ 2 -test), and an additional reduction was evident among both the IgM- and IgG-expressing memory B-cell populations ( P <0.001; χ 2 –test; Fig. 6d ). However, the pattern in IgG-expressing splenic and bone marrow plasma cells was more alike the IgG + GC B cells, albeit with significant differences ( P <0.001; χ 2 -test; Fig. 6e , and Supplementary Figs 9a,b and 10a ). Thus, this showed that in SLC −/− mice, cells expressing a H chain with a prototypic ANA H-CDR3 had an advantage in order to enter but not to exit the GC compartment, and suggested different selection thresholds to enter the memory B-cell and plasma cell pools. Clonal selection based on H-CDR3 To further investigate the selection in the GCs, the H-CDR3 sequences were analysed for length and identity. In the naive B cells from SLC −/− mice, the H-CDR3 sequences showed a length distribution that appeared normal with an average of 12 aa residues and, as may be expected of naive B cells, the vast majority was different ( Fig. 6f ), demonstrating a polyclonal repertoire. The pattern in IgM + GC B cells was very different, and although the lengths of the H-CDR3 varied also in this population, some were more frequent, for example, those with 11 and 12 aa residues. Moreover, the vast majority of H-CDR3 sequences of a particular length, for example, 11 aa residues, was identical. This was also evident in the IgG-expressing GC B and spleen plasma cells, although clones with a shorter H-CDR3, for example, 7 aa residues, were more frequent ( Fig. 6f,g ). This became even more evident in the memory B-cell populations, with a dominance of either 6 and 12 or 6 and 14 aa residues in length in the IgM + and IgG + memory populations, respectively. Thus, this suggests that in SLC −/− mice, the H-CDR3 sequence is critical in GC selection, with the strongest selection pressure on GC B cells that enter the memory B-cell pools. Exclusion of V H 81X from the memory B-cell and plasma cell pools During our sequence analyses, we noticed that V H 81X ( V H 5-2 ) usage was sequentially enriched from ∼ 0.5% among the naive B cells to 2% in the IgM + and 15% in the IgG + GC B-cell pools from SLC −/− mice ( P <0.001; χ 2 -test; Fig. 7a ). V H 81X is one of the most well-studied mouse V H genes, as it is intrinsically self-reactive, overrepresented early in ontogeny and found in natural autoantibodies, as well as in mouse lupus models [21] , [47] , [48] , [49] . In adult mice, V H 81X usage is high in pro-B but low in naive B cells [50] , and as it was low also in the naive B cells from SLC −/− mice, we were surprised by its enrichment among the GC B cells. Analysing the V H 81X sequences showed a sequential enrichment for J H 3 , from ∼ 30% in the naive to 80% in the IgG + GC B cells ( Fig. 7b ), and a sequential reduction in H-CDR3 length from 12 to 8 aa residues in the IgG + GC B cells ( Fig. 7c ), consistent with clonal selection. Moreover, the proportion of V H 81X sequences with a prototypic H-CDR3 followed a pattern similar to that of the entire V H repertoire with an enrichment among the IgM + and reduction among the IgG + GC B cells ( Figs 7d and 6d ). 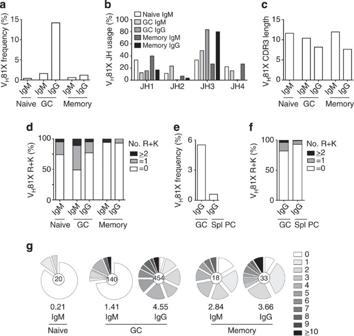Figure 7: Expansion ofVH81X-expressing B cells in GC but exclusion from the memory B-cell and plasma cell pools. (a–g) Analysis ofVH81Xsequences in naive B, GC B-cell, memory B-cell and splenic (Spl) plasma cell (PC) populations inSLC−/−mice. (a)VH81Xusage in indicated cell populations. (b)JHusage and (c) H-CDR3 length inVH81Xsequences in indicated cell populations. (d) Proportions of H-CDR3 sequences with 0, 1 or ≥2 arginine (R) and/or lysine (K) residues in indicated cell populations. (e)VH81Xusage in indicated cell populations. (f) Proportions of H-CDR3 sequences with 0, 1 or ≥2 arginine (R) and/or lysine (K) residues in indicated cell populations. (g) Sequence analysis of expressedVH81Xgenes in sorted naive, GC and memory B cells. Pie charts show the proportions ofVH81Xsequences that carry 1, 2, 3 and so on point mutations in indicated cell populations. The number below shows the average number of mutations perVH81X. Data are from a pool of six (a–d,g) and five (e,f)SLC−/−mice. The number ofVH81Xsequences analysed are at the pie chart centre. Figure 7: Expansion of V H 81X -expressing B cells in GC but exclusion from the memory B-cell and plasma cell pools. ( a – g ) Analysis of V H 81X sequences in naive B, GC B-cell, memory B-cell and splenic (Spl) plasma cell (PC) populations in SLC −/− mice. ( a ) V H 81X usage in indicated cell populations. ( b ) J H usage and ( c ) H-CDR3 length in V H 81X sequences in indicated cell populations. ( d ) Proportions of H-CDR3 sequences with 0, 1 or ≥2 arginine (R) and/or lysine (K) residues in indicated cell populations. ( e ) V H 81X usage in indicated cell populations. ( f ) Proportions of H-CDR3 sequences with 0, 1 or ≥2 arginine (R) and/or lysine (K) residues in indicated cell populations. ( g ) Sequence analysis of expressed V H 81X genes in sorted naive, GC and memory B cells. Pie charts show the proportions of V H 81X sequences that carry 1, 2, 3 and so on point mutations in indicated cell populations. The number below shows the average number of mutations per V H 81X . Data are from a pool of six ( a – d , g ) and five ( e , f ) SLC −/− mice. The number of V H 81X sequences analysed are at the pie chart centre. Full size image By contrast to the GC B cells, those expressing V H 81X were in principal excluded (1%) from both the IgM + and IgG + memory pools ( Fig. 7a ). Analysing those that did enter, based on J H 3 usage and H-CDR3 length, the V H 81X -expressing IgG + memory B cells clearly originated from the IgG + GC B cells, whereas the IgM + memory cells were reminiscent of the naive B cells ( Fig. 7b,c ). Further, V H 81X sequences with a prototypic ANA H-CDR3 were almost absent from the memory pools ( Fig. 7d ). Cells expressing V H 81X were also excluded from the spleen and BM plasma cell pools ( Fig. 7e and Supplementary Fig. 10b ), and among the few V H 81X -expressing plasma cells a reduction in those with a prototypic ANA H-CDR3 was evident in the spleen ( Fig. 7f ), but not in the BM ( Supplementary Fig. 10c ). Nevertheless, a lack of V H 81X -expressing cells in both the memory B-cell and plasma cell pools could potentially be explained by these cells remaining in the GCs, and presumably continue to undergo SHM. However, the V H 81X sequences in the GC B cells displayed fewer mutations per V H sequence than those in the entire V H repertoire ( Figs 7g and 6c ), observed also in the plasma cell but not IgG memory B-cell pool ( Figs 7g and 6c , and Supplementary Fig. 10d,e ). Thus, as most of the cells expressing V H 81X do not exit the GCs, and as they do not accumulate a large number of mutations, V H 81X -expressing cells seemingly undergo deletion in the GCs. That B cells expressing V H 81X , a BCR with an intrinsically self-reactive V H , are expanded in the GCs in SLC −/− mice but excluded from the memory B and plasma cell pools support the hypothesis that peripheral B-cell tolerance in these mice is maintained by selection thresholds on cells entering the memory B-cell and plasma cell pools. The absence of SL chain allows the development of self-reactive naive B cells, which is sufficient to drive the spontaneous formation of persistent autoreactive Td GCs. Interestingly, peripheral tolerance appears maintained by selection thresholds on the GC B cells entering into the memory B-cell and plasma cell pools. Although some do enter the short-lived plasma cell pool and produce IgG ANAs, those that express seemingly more autoreactive BCRs, for example, the intrinsically self-reactive V H 81X in combination with an ANA H-CDR3, are excluded. Even though this in itself is not sufficient to tip the balance to overt autoimmunity, it could potentially result in the production of pathogenic autoantibodies. In current models of B-cell development, some degree of autoreactivity displayed by the pre-BCR appears to be critical for downstream signalling events at the pre-B-cell stage [24] , [25] , [26] , [27] , [51] . This is provided by the λ5-tail that interacts with molecules on stromal cells and with neighbouring μH chains [24] , [26] , [52] , [53] . The autoreactivity model is supported by studies in λ5T mice, where expression of a transgenic BCR ( 3–83 ) is sufficient to rescue the development of normal B-cell numbers, but only in the presence of autoantigen [54] . Provided that there is a requirement for an autoreactive receptor, pre-BCR or μH chain, this would imply that a majority of pre-B cells in SLC −/− mice express a μH chain with some degree of autoreactivity. As we show here, pre-B cells in SLC −/− mice are indeed enriched for those that express a prototypic ANA H-CDR3. However, selection at subsequent stages ensures that the proportion of such cells is reduced in the FO B-cell pool. Nevertheless, this pool is still enriched for self-reactivity, which is supported by the spontaneous formation of GCs with an even higher proportion of IgM + B cells that also express μH chains with a prototypic ANA H-CDR3. In humans, usage of the autoreactive 9G4 idiotype in the naive B-cell pool of SLE patients is not different from that of healthy individuals and RA patients [55] , [56] . However, owing to its expansion in GCs, and exit into the memory B and long-lived plasma cell pools, 9G4 autoantibodies are abundant in SLE patients, whereas in healthy subjects and RA patients B cells expressing the 9G4 idiotype are not even allowed to enter GCs [55] . Spontaneous formation of Td GCs is observed also in mouse lupus models [14] . Among B-cell hybridomas with anti-DNA/ANA reactivity established from lupus mice, V H 81X usage is higher than expected [21] , [47] . It would thus appear that this particular H chain is undesirable in GCs as well as in the long-lived memory B-cell and plasma cell pools, that is, under conditions where SHMs could give rise to pathogenic autoantibodies. By analogy to 9G4 + cells, V H 81X usage in the naive B cells from SLC −/− mice is not different from that of controls, and is consistent with observations in λ5T mice [57] . However, despite its normal usage in the naive pool, B cells expressing this particular V H enter and expand in the GCs in SLC −/− mice. By contrast to 9G4 though, V H 81X and especially in combination with a prototypic ANA H-CDR3 is, in principal, excluded from both the memory B-cell and plasma cell pools in SLC −/− mice. Also GC B cells that express other V H genes with a prototypic ANA H-CDR3 follow a similar pattern, although selection on those entering the plasma cell pool is not as strong consistent with the production of IgG2b/c ANAs by short-lived plasma cells. The apparent counter-selection of autoreactivity in the GCs support the hypothesis that peripheral B-cell tolerance in these mice is maintained by different selection thresholds on cells entering the memory B-cell and plasma cell pools. Analyses of anti-DNA and ANAs from mouse lupus models and SLE patients have shown that they are clonally related and have undergone SHM, hence derive from a typical Td GC response [15] , [21] , [55] . It has also been found that reverting these mutations to the germline sequence abolishes antigen binding [10] , [15] , [58] , which has led to a model where de novo mutations in GCs give rise to autoreactivity. Under normal circumstances, autoreactive B cells would undergo deletion, whereas in disease situations failure to induce tolerance in GCs would allow such cells to survive. Indeed, de novo mutations in GCs can lead to high-affinity autoantibody production, provided the antigen is not present in the GCs [10] . However, this does not exclude that naive B cells expressing self-reactive BCRs, for example, 9G4 in SLE or those described in RA patients [1] , [2] , [55] , act as initiators of GC formation, by analogy to, for example, V H 81X , as we show here. It has been shown that, for example, viruses can induce autoantibody production [59] , and although a germ-free environment does not affect disease severity in a lupus model, a change in diet results in a milder disease [35] . As the antigen(s) that initially activates the naive B cells in SLC −/− mice is unknown, it could be self-antigen, although we cannot exclude that it is an antigen not depleted by the antibiotics treatment, for example, food antigens, viruses or remaining microbes. A mutant Roquin protein causes dysregulation of T FH cells resulting in excessive numbers of GCs and disease [60] . It has also been proposed that there is a link between overstimulation of T FH cells and the development of dysregulated antibody responses [61] . In the SRBC-immunized mice and mouse models of autoimmune diseases, T FH cells are found in limiting numbers in the GCs [14] , whereas in the GCs in the SLC −/− mice there is an excess of T FH cells. In the latter, B-cell proliferation and survival are also different, and perhaps this ‘excess’ of T FH cells is a means to ensure that the B cells exiting the GCs do not express high-affinity autoantibodies. Most autoimmune diseases are multigenic, suggesting that multiple mutations, inherited and somatic, are required for disease development. This is also consistent with the detection of autoantibodies long before disease onset in, for example, RA and SLE patients [6] , [7] , implicating the development of self-reactive naive B cells as a predisposing factor. However, to tip the balance to manifest disease, which may take years or decades, additional factors would be required, either genetic and/or, for example, immunological triggers. A number of genes and loci have been associated with these diseases affecting, for example, (1) B-cell signalling pathways, (2) phagocytosis of apoptotic cells and (3) the interferon and TLR pathways [62] . Hence, the SLC −/− mouse can serve as a model in which to explore the effect of additional factors. Although it is not known whether a dysfunctional SL chain predisposes to autoimmune disease, copy number variation in VPREB1 has been associated with clinical parameters in RA patients [63] . Mice The SLC −/− mice [64] , previously backcrossed for ≥10 generations on the C57BL/6OlaHsd background, were after embryo transfer bred onto the C57BL/6NCrl background and then intercrossed to establish SLC −/− mice. Mice were kept in the Gothenburg University specific pathogen free animal facility under project licence authorization (245–2009, 330–2012 and 39–2010) approved by the local ethics committee, and experiments were performed in compliance with ethical regulations. Mice were genotyped by PCR for targeting of VpreB2 and VpreB1 / λ5 (ref. 64 ). Control mice (C57BL/6NCrl) were purchased from Charles River Laboratories(Germany) and Taconic (Denmark). Female mice were used throughout, aged 1–11 months. Flow cytometry Single-cell suspensions were stained with a cocktail of monoclonal antibodies, ( Supplementary Table 4 ) following standard techniques, and permeabilization buffers according to manufacturer’s instructions, and were analysed on FACSCantoII, FACSVerse (BD Biosciences) or Synergy (Sony Biotechnology) flow cytometers. Data were analysed using FlowJo software (Treestar Inc.). Owing to the high proportion of B1 B cells among the CD21 − 23 − population on the C57BL/6NCrl compared with the C57BL/6OlaHsd background [28] , these (CD43 + ) were excluded in the analysis. Cell sorting BM and spleen cells were collected and enriched for B cells using CD19 MACS beads (Miltenyi Biotec), followed by sorting pro-B (B220 + c-kit + ), pre-B (B220 + c-kit − CD25 + ), immature (B220 + CD93 + IgM + ) and FO (B220 + CD93 − 43 − 21 int 23 + ) B cells. T FH cells (CD4 + PD-1 hi ) and naive CD4 + T cells (CD4 + PD-1 − ) were sorted from individual SLC −/− mice. Sort 1 ( Figs 6 and 7 ): spleen cells were collected from SLC −/− mice followed by sorting GC (B220 + GL7 + CD95 + ), naive (B220 + CD93 − 43 − 80 − PD-L2 − 73 − ) and memory (B220 + CD93 − 43 − 80 + PD-L2 + 73 + ) B cells. Sort 2 ( Figs 6 and 7 , and Supplementary Fig. 9 ): spleen GC B and plasma cells, and BM plasma cells were sorted from a pool of five SLC −/− mice. GC B and plasma cells were obtained by enrichment-sort for CD19 + CD93 − and CD19 low/+ CD93 hi cells, followed by purity-sort for GC B (CD19 + CD95 + GL7 + ) and plasma (CD19 low/+ CD93 hi ) cells. BM plasma cells were obtained by enrichment-sort for B220 − CD138 hi cells, followed by purity-sort using the same markers ( Supplementary Fig. 9 ). Cells were sorted on a FACSAria (BD Biosciences) or Synergy cell sorter (Sony Biotechnology) with purities >90%. Immunohistochemistry Spleens of SLC −/− and control mice were collected and embedded in OCT compound (TissueTek, Tokyo, Japan), snap-frozen in liquid nitrogen and stored at −80 °C. Intestine was collected from SLC −/− mice that had undergone antibiotics treatment. Frozen sections (8 μm) were cut using a cryostat Leica, (Wetzlar, Germany) and stained ( Supplementary Table 4 ). For intracellular staining of Bcl-6 and Ki-67, the sections were permeabilized using PBS with 0.1% saponin before blocking with normal horse serum. Subsequently, the sections were stained for 30–60 min at room temperature with primary antibody except for Bcl-6, which was stained overnight at 4 °C. Images were acquired using LSM 700 confocal microscope and ZEN 2009 acquisition software (Zeiss). Reverse transcription and qPCR RNA was isolated using RNeasy kit (Qiagen) and cDNA was reversely transcribed using SuperScript II (Invitrogen). Aicda was quantified by qPCR and normalized to the expression of Gapdh (Applied Biosystems), and cDNA from Peyer’s patches was used as positive control. Primer sequences are described in Supplementary Table 5 , and Power SYBR Green was used (Applied Biosystems). For gene profiling of FO B cells, the cDNA was applied to TaqMan RT-PCR Mouse Immune Array microfluidic cards (47365297; Applied Biosystems) and data were analysed as described in the manufacturer’s protocol. All samples were run in triplicates on a ViiA7 system and analysed with the ViiA7 basic software (Applied Biosystems). Immunizations SRBCs in sterile Alsever’s solution were purchased from the National Veterinary Institute (HåtunaLab, Bro, Sweden) and stored at 4 °C. SRBCs were washed in PBS three times before immunizing control mice with 5 × 10 8 cells in 0.2 ml PBS in the tail vein [65] . Antibiotic treatment Three- to four-week-old SLC −/− mice were treated with broad-spectrum antibiotics in drinking water over 4 weeks starting at the day of weaning. Antibiotics: vancomycin (500 mg l −1 ), nebcina (30 mg l −1 ), metronidazole (1 g l −1 ) dissolved in NaCl and ampicillin (1 g l −1 ). Sucrose and 0.2% NaCl (because of the metronidazole) was added to the water. Anti-CD40L treatment SLC −/− mice were treated at days 0, 2 and 4 with anti-CD40L or control hamster Ig (BioXCell), 250 μg per injection intravenously. Mice were either killed on day 6 or treated with an additional injection of 500 μg on day 11 and then killed 5 weeks post the first injection. HEp2-assay Serum ANAs were detected using HEp2 cell-coated slides (Bio-Rad Laboratories) [28] . Serum was diluted 1:40 or serially diluted ( Fig. 5i ) before incubating on the slides for 30 min at RT, then washed in PBS and visualized with Alexa Fluor 488-conjugated goat anti-mouse IgG2b (Invitrogen) or IgG2c antibodies (Jackson ImmunoResearch). Sera from a pool of age-matched C57BL/6NCrl mice were used as negative control. Confocal fluorescence images were captured with a LSM 700 confocal microscope and ZEN 2009 acquisition software (Zeiss). Two independent observers assessed the intensity of the staining. Apoptosis assay After surface staining, apoptotic cells were detected by incubation with zVAD-FMK-FITC (CaspGlow, eBioscience) in RPMI 1640 for 1 h at 37 °C, according to manufacturer’s protocol and then analysed by flow cytometer. High-throughput sequencing of Ig genes RNA was isolated using RNeasy kit (Qiagen) and cDNA synthesis was performed according to the SuperScript II RT protocol (Invitrogen). The forward MsVHE primer, representing a consensus sequence of highly conserved codons at the beginning of FWR1, was combined with reverse primers [66] ( Supplementary Table 5 ), amplifying Igμ and Igγ transcripts independently with 10 base multiplex identifier tails. To produce sufficient amounts of DNA for sequencing, while minimizing PCR amplification, 30 cycles were performed using Phusion High-Fidelity DNA Polymerase (NEB). PCR products were purified using QIAquick Gel Purification Kit. Purified samples were mixed in equal quantities for sequencing on the GS FLX+ Titanium or GS Junior+ sequencer at Eurofins MWG Operon (Germany). Sequences were assigned to the corresponding samples based on the multiplex identifier tags. After passing the quality control criteria, sequences were submitted to IGMT/HighV-QUEST database for analysis [67] . The files from IMGT/highV-QUEST were imported into IgAT immunoglobulin analysis tool for further analysis [68] . Statistics Mean values and s.e.m. are displayed in the plots. P values were calculated using appropriate statistical test: paired and unpaired t -test (GraphPad Prism), or χ 2 -test (SPSS). * P <0.05, ** P <0.01, *** P <0.001. Accession code. The sequencing data are deposited in NCBI Sequence Read Archive (SRA) under the BioProject PRJNA277306 (accession code: SRP055855 ). How to cite this article: Grimsholm, O. et al . Absence of surrogate light chain results in spontaneous autoreactive germinal centres expanding V H 81X -expressing B cells. Nat. Commun . 6:7077 doi: 10.1038/ncomms8077 (2015).